The fourth crystallographic closest packing unveiled in the gold nanocluster crystal Metal nanoclusters have recently attracted extensive interest not only for fundamental scientific research, but also for practical applications. For fundamental scientific research, it is of major importance to explore the internal structure and crystallographic arrangement. Herein, we synthesize a gold nanocluster whose composition is determined to be Au 60 S 6 (SCH 2 Ph) 36 by using electrospray ionization mass spectrometry and single crystal X-ray crystallography (SCXC). SCXC also reveals that Au 60 S 6 (SCH 2 Ph) 36 consists of a fcc-like Au 20 kernel protected by a pair of giant Au 20 S 3 (SCH 2 Ph) 18 staple motifs, which contain 6 tetrahedral-coordinate μ 4 -S atoms not previously reported in the Au–S interface. Importantly, the fourth crystallographic closest-packed pattern, termed 6H left-handed helical (6HLH) arrangement, which results in the distinct loss of solid photoluminescence of amorphous Au 60 S 6 (SCH 2 Ph) 36 , is found in the crystals of Au 60 S 6 (SCH 2 Ph) 36 . The solvent-polarity-dependent solution photoluminescence is also demonstrated. Overall, this work provides important insights about the structure, Au–S bonding and solid photoluminescence of gold nanoclusters. Bridging gold atom (or gold complexes) [1] , [2] , [3] and nanocrystals (typically >3 nm) [4] , [5] , [6] , [7] , [8] , gold nanoclusters [9] , [10] , [11] , [12] , [13] , [14] , [15] have recently attracted increasing research interest due to their well-defined compositions and structures, unique properties and potential applications. In particular, the structures of gold nanoclusters are of primary significance and have received the most extensive attention in the research community [16] , [17] , [18] , [19] , [20] , [21] . However, structure achievements remain limited due to the difficulty of precise size control and structural resolution, especially for relatively large gold nanoclusters [22] , [23] , [24] , [25] , [26] . It is generally believed that the gold nanoclusters adopt kernel-staple structures, and the staple motifs play a vital role in stabilizing the nanoclusters. The large staple motif Au 8 (SR) 8 was reported in Au 20 (SR) 16 nanocluster [27] , but the question remains whether there is a larger staple motif. Although thiolate or sulfido (-S-) can be found in the surface of gold nanoclusters as protecting ligands, both thiolate sulfur and sulfido (-S-) are always three-coordinate (mainly μ 2 -S and rarely μ 3 -S) [28] , [29] , naturally raising the question of whether there are sulfurs with any other coordination numbers in gold nanoclusters. Notably, four-coordinate μ 4 -S and five-coordinate μ 4 -S have been reported in Cr(III) and Cu(I) complexes [30] , [31] , respectively, but such high-coordinate sulfur has not been found in Au–S interfaces (not limited to gold nanoclusters). In addition to these internal structure questions, there are some other crystallographic arrangement issues that need to be addressed. It is known that there are two classic crystallographic closest packings for atomic crystals: the fcc arrangement with a packing sequence of ‘ABC’ found in bulk Au, Ag, Pd, Pt and Ir metals [32] , FePt nanoparticles [33] , and others; and the hcp or 2H arrangement with a packing sequence of ‘AB’ revealed in Rh nanosheets [34] , Au square sheets [35] , PbPt nanorods [36] , BiPt nanoplates [37] , among others. The third closest packing, named the 4H arrangement, has a packing sequence of ‘ABCD’ and was first observed in bulk Ag by Novgorodova et al . in 1979 (ref. 38 ), then subsequently revealed in Ag nanocrystals and nanowires [39] , [40] , Au nanoribbons [41] and more. The advances in gold nanocluster research provide opportunities to discover novel closest-packed patterns. It is worth noting that in contrast to gold nanocrystals, molecule-like gold nanoclusters can grow high-quality single crystals for X-ray crystallography analyses. Thus, not only the internal structure (atom packing in every gold nanocluster) but also the crystallographic arrangement (the arrangement of gold nanoclusters in single crystals) of gold nanoclusters can be resolved by single crystal X-ray crystallography (SCXC). Jin et al . reported the fcc crystallographic arrangement of Au 30 (SR) 18 nanoclusters in early 2016 (ref. 42 ), and very recently, Wu et al . reported the 4H crystallographic arrangement in Au 92 crystals [43] . It is currently unknown whether there are any other intriguing arrangement patterns in gold nanoclusters. To address this question, together with the above mentioned issues, more gold nanoclusters with complex surfaces must be synthesized, and their structures must be resolved. Herein, we report the synthesis, structure (including internal and crystallographic) and photoluminescence of a gold nanocluster whose composition is determined to be Au 60 S 6 (SCH 2 Ph) 36 using electrospray ionization mass spectrometry (ESI-MS) and SCXC. In particular, we find a fourth closest packing in the crystal of Au 60 S 6 (SCH 2 Ph) 36 . Synthesis and characterization The Au 60 S 6 (SCH 2 Ph) 36 nanocluster was obtained via a thermal-induced ligand exchange reaction of molecularly pure Au 38 (SC 2 H 4 Ph) 24 with excess phenylmethanethiol (HSCH 2 Ph). Of note, the interesting thing in this synthesis is that the protecting ligand of the starting nanoclusters and the incoming ligand only have subtle difference in composition (-CH 2 -, see Supplementary Fig. 1 ), which may have some implications to other nanoparticles (including quantum dots) synthesis. Briefly, the reaction was initialized by dissolving 10 mg of Au 38 (SC 2 H 4 Ph) 24 nanoclusters in 1 ml of toluene containing 0.5 ml of HSCH 2 Ph, with stirring. After proceeding overnight at 100 °C under nitrogen atmosphere, the reaction was terminated by the addition of plenty of methanol. The crude product was thoroughly washed with petroleum ether and methanol for four times, then subjected to subsequent separation and purification by preparative thin-layer chromatography (PTLC) [19] . Single crystals of the purified nanoclusters were grown by the vapour diffusion of acetonitrile into the toluene solution of the purified nanoclusters at 5 °C. Black-coloured crystals were formed after one week. As shown in Fig. 1a , the optical absorption spectrum of the as-obtained nanocluster has no dominant visible absorption peak and only shows a very weak absorption at ∼ 345 nm (3.59 eV) and a step at ∼ 600 nm (2.07 eV). The optical energy gap was determined to be ∼ 1.73 eV by extrapolating the lowest-energy absorption peak to zero absorbance (see the inset in Fig. 1a ). The composition of the as-obtained nanocluster was identified by ESI-MS. Of note, without the addition of cesium acetate (CsOAc), no signal was observed in either positive or negative mode, which implies the charge neutrality of the nanocluster. To impart charges, CsOAc was added to the nanocluster solution to form positively charged [cluster+ x Cs] x + adducts in the electrospray process. As shown in Fig. 1b , two intense peaks at mass/charge ratio ( m/z ) 8,356.22 and 5,615.49 are observed, which can be readily assigned to [Au 60 S 6 (SCH 2 Ph) 36 Cs 2 ] 2+ (calculated: 8,356.31, deviation: 0.09) and [Au 60 S 6 (SCH 2 Ph) 36 Cs 3 ] 3+ (calculated: 5,615.51, deviation: 0.02), respectively. Thus, the as-obtained nanocluster should be Au 60 S 6 (SCH 2 Ph) 36 , which was further confirmed by the subsequent SCXC analysis. 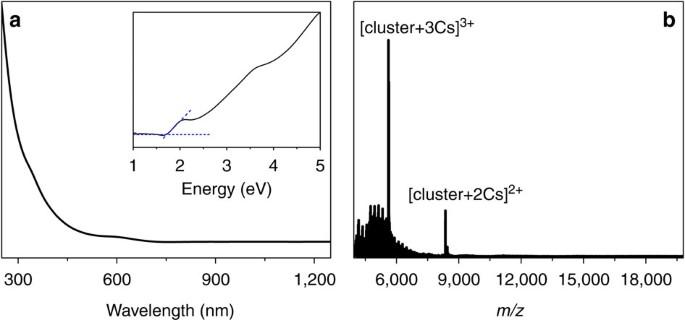Figure 1: Characterization of Au60S6(SCH2Ph)36. Ultraviolet-visible-near-infrared spectrum (a) and electrospray ionization mass spectrometry (ESI-MS) (positive ion mode) spectrum (b) of Au60S6(SCH2Ph)36. The inset ofarepresents the spectrum on the energy scale. Figure 1: Characterization of Au 60 S 6 (SCH 2 Ph) 36 . Ultraviolet-visible-near-infrared spectrum ( a ) and electrospray ionization mass spectrometry (ESI-MS) (positive ion mode) spectrum ( b ) of Au 60 S 6 (SCH 2 Ph) 36 . The inset of a represents the spectrum on the energy scale. Full size image Internal structure The structure of the as-obtained nanocluster was determined by SCXC. 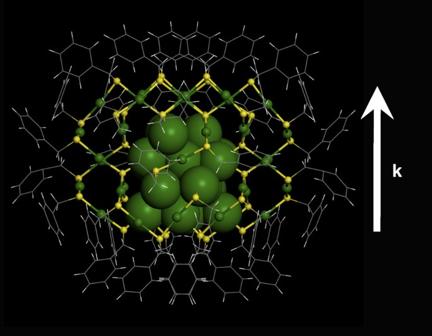Figure 2: X-ray atomic structure of the Au60S6(SCH2Ph)36nanocluster. The Au atoms are in green, the sulfur atoms are in yellow, and the benzyls are in wireframe. The vertical upward arrow indicates the direction of thek-vector. Figure 2 presents the total structure of the as-obtained nanocluster, which crystallizes in a hexagonal P 6522 space group, has no centre or plane of symmetry and only possesses a C 2 rotation axis of symmetry. The as-obtained nanocluster consists of an Au 20 kernel and a pair of giant Au 20 S 3 (SCH 2 Ph) 18 staple motifs. The Au 20 kernel can be viewed as a fragment of the fcc structure in bulk gold or nanoparticles, typically >3 nm (diameter). The 16 gold atoms in the kernel constitute an Au 16 tetrahedron without vertex ( Fig. 3a,e ), and each facet of the tetrahedron is a distorted hexagon. The other 4 Au atoms (highlighted in blue and red, Fig. 3b,f ) in the kernel are capped on the four facets of the tetrahedron in a one-to-one fashion. Moreover, the Au 20 kernel is protected by a pair of giant unanimous Au 20 S 3 (SCH 2 Ph) 18 staple motifs: one Au 20 S 3 (SCH 2 Ph) 18 staple connects to the Au 20 kernel ( Fig. 3c,g ; the back view can be found in Supplementary Fig. 2 ) by five terminal μ 2 -S atoms (binding to one kernel Au atom, one staple Au atom and one -CH 2 Ph group, indicated by white arrow, see Fig. 3i,j ) and three bridging μ 4 -S atoms (binding to one kernel Au atom and three staple Au atoms, highlighted in the white circle, see Fig. 3i,j ), and the other Au 20 S 3 (SCH 2 Ph) 18 staple binds to the Au 20 kernel in the same fashion after rotating (180°) along the C 2 axis of symmetry ( Fig. 3d,h ). It is worth noting that in addition to the common three-coordinate μ 2 -S atoms (binding to one R group and two Au atoms (Au–SR–Au), see Fig. 3k ), there are six tetrahedral-coordinate S atoms ( μ 4 -S) (every μ 4 -S binds to four Au atoms, see Fig. 3l ), indicating the uniqueness of Au–S bonding in the Au 60 S 6 (SCH 2 Ph) 36 nanocluster. Herein, the six surprising μ 4 -S atoms should come from the thiol, which may undergo S–C bond cleavage under heating conditions during the ligand-exchange-induced structure transformation process [42] . A single Au 20 S 3 (SR) 18 staple motif (branched at the site of the μ 4 -S atom) contains two -Au-SR-Au- and three -Au-SR-Au-SR-Au- units between the five terminal μ 2 -S atoms and three bridging μ 4 -S atoms, and one -Au-SR-Au-SR-Au- and one -Au-SR-Au-SR-Au-SR-Au- units among the three bridging μ 4 -S atoms ( Fig. 3j ). Of note, such a giant staple motif has not been found in thiolated gold nanoclusters, which is larger than the Au 8 (SR) 8 staple motif in Au 20 (SR) 16 nanoclusters [27] . Figure 2: X-ray atomic structure of the Au 60 S 6 (SCH 2 Ph) 36 nanocluster. The Au atoms are in green, the sulfur atoms are in yellow, and the benzyls are in wireframe. The vertical upward arrow indicates the direction of the k -vector. 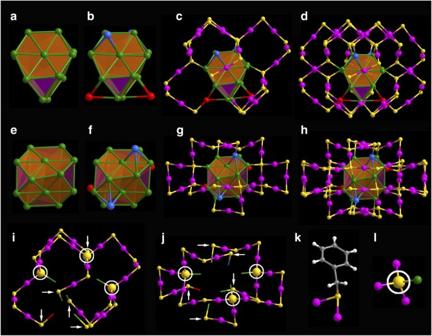Figure 3: Anatomy of the atomic structure of Au60S6(SCH2Ph)36nanocluster. (a,e) Side and top view of the Au16tetrahedron without vertex; (b,f) side and top view of Au20inner kernel; (c,g) side and top view of Au20kernel with an Au20S3(SCH2Ph)18staple motif; (d,h) side and top view of the overall framework of the Au60S6(SCH2Ph)36nanocluster with a pair of Au20S3(SCH2Ph)18staple motifs; (i,j) side and top view of the Au20S3(SCH2Ph)18staple motif; (k) theμ2-S atom and (l) theμ4-S atom (highlighted in the white circle). Colour labels: yellow=S, white=H, gray=C, other colour=Au. The Au atoms are represented in different colours to differentiate from them each other on the bonding ways and occupying positions. Full size image Figure 3: Anatomy of the atomic structure of Au 60 S 6 (SCH 2 Ph) 36 nanocluster. ( a , e ) Side and top view of the Au 16 tetrahedron without vertex; ( b , f ) side and top view of Au 20 inner kernel; ( c , g ) side and top view of Au 20 kernel with an Au 20 S 3 (SCH 2 Ph) 18 staple motif; ( d , h ) side and top view of the overall framework of the Au 60 S 6 (SCH 2 Ph) 36 nanocluster with a pair of Au 20 S 3 (SCH 2 Ph) 18 staple motifs; ( i , j ) side and top view of the Au 20 S 3 (SCH 2 Ph) 18 staple motif; ( k ) the μ 2 -S atom and ( l ) the μ 4 -S atom (highlighted in the white circle). Colour labels: yellow=S, white=H, gray=C, other colour=Au. The Au atoms are represented in different colours to differentiate from them each other on the bonding ways and occupying positions. Full size image Crystallographic arrangement Interestingly, Au 60 S 6 (SCH 2 Ph) 36 nanoclusters adopt the closest packing, and a very special stacking sequence of ‘ABCDEF’ along the close-packed [001] direction is found in its single crystals ( Fig. 4a ). The Au 60 S 6 (SCH 2 Ph) 36 nanoclusters in every stacking layer ((001) plane) are arranged uniformly, and each nanocluster is surrounded by six identical nanoclusters with the same tropism ( k -vector), as shown in Fig. 4b and Supplementary Fig. 3 . Moreover, the stacking layer perpendicular to the [001] direction can overlap completely with its neighboring layer after every nanocluster in the layer rotates (60°) clockwise or anti-clockwise along the z axis ( Supplementary Fig. 3 ), and thus the arrangement of Au 60 S 6 (SCH 2 Ph) 36 nanoclusters in single crystals along the [001] direction is reminiscent of the left-handed helix ( Supplementary Fig. 4 ). For clarity, a left-handed helical sequence, here termed the 6H left-handed helical (6HLH) arrangement, is isolated from the crystal, as shown in Fig. 4c,d . Such a crystallographic arrangement is not only interesting but also exciting, as the third closest packing in crystals, named 4H, was found in 1979 (ref. 38 ). 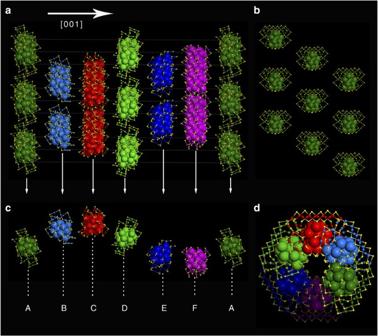Figure 4: 6HLH crystallographic arrangement of Au60S6(SCH2Ph)36nanoclusters. (a) The stacking sequence along the [001] direction; (b) the closest-packed pattern of Au60S6(SCH2Ph)36nanoclusters in the (001) plane; (c,d) different views of the left-handed helical arrangement of Au60S6(SCH2Ph)36nanoclusters. (Note: to highlight the 6HLH arrangement, the Au atoms of the nanoclusters in each close-packed plane are labeled in different colours). Figure 4: 6HLH crystallographic arrangement of Au 60 S 6 (SCH 2 Ph) 36 nanoclusters. ( a ) The stacking sequence along the [001] direction; ( b ) the closest-packed pattern of Au 60 S 6 (SCH 2 Ph) 36 nanoclusters in the (001) plane; ( c , d ) different views of the left-handed helical arrangement of Au 60 S 6 (SCH 2 Ph) 36 nanoclusters. (Note: to highlight the 6HLH arrangement, the Au atoms of the nanoclusters in each close-packed plane are labeled in different colours). Full size image Photoluminescence The 6HLH arrangement indicates the unique interactions among Au 60 S 6 (SCH 2 Ph) 36 nanoclusters in the single crystals, which is supported by the photoluminescence intensity comparison between the amorphous and crystallized Au 60 S 6 (SCH 2 Ph) 36 as shown in Fig. 5 . Although the emission spectrum profiles of the disordered (amorphous) Au 60 S 6 (SCH 2 Ph) 36 is almost superimposable to that of the ordered (crystallized) Au 60 S 6 (SCH 2 Ph) 36 , the emission intensity of the former is ∼ 1.7 folds of that of the latter. The lower photoluminescence intensity in crystallized Au 60 S 6 (SCH 2 Ph) 36 might be caused by the energy transfer among the 6HLH arranged Au 60 S 6 (SCH 2 Ph) 36 nanoclusters, indicating the notable interactions among the 6HLH arranged Au 60 S 6 (SCH 2 Ph) 36 nanoclusters. Although the 6HLH arrangement barely changes the emission spectrum, solvent does result in the obvious blue-shift of the maximum emission peak, and interestingly, the blue-shift increases with the increase of solvent polarity, while the photoluminescence intensity of Au 60 S 6 (SCH 2 Ph) 36 nanoclusters decreases with the increase of solvent polarity (see Fig. 6 ). Anyway, these facts indicate that the solution photoluminescence of Au 60 S 6 (SCH 2 Ph) 36 is solvent-polarity dependent. 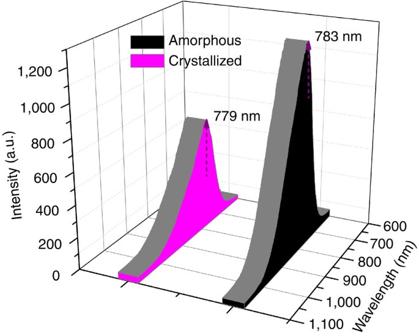Figure 5: The solid photoluminescence spectra of Au60S6(SCH2Ph)36nanoclusters. Au60S6(SCH2Ph)36nanoclusters in crystallized and amorphous states exhibit obviously different photoluminescence intensities but almost identical emission spectrum profiles. Note: the excitation wavelengthλex=514 nm. Figure 5: The solid photoluminescence spectra of Au 60 S 6 (SCH 2 Ph) 36 nanoclusters. Au 60 S 6 (SCH 2 Ph) 36 nanoclusters in crystallized and amorphous states exhibit obviously different photoluminescence intensities but almost identical emission spectrum profiles. Note: the excitation wavelength λ ex =514 nm. 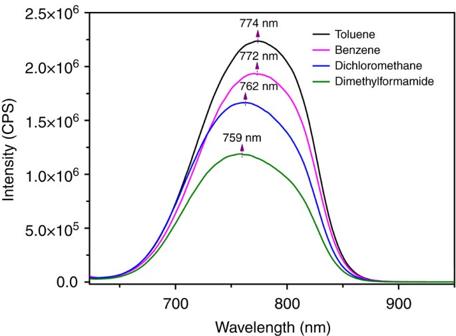Figure 6: The solvent-polarity-dependent solution photoluminescence of Au60S6(SCH2Ph)36nanoclusters. Not only the maximum emission wavelengths but also the photoluminescence intensities of Au60S6(SCH2Ph)36nanoclusters in solution are dependent on the solvent polarity. Note: the excitation wavelengthλex=514 nm. Full size image Figure 6: The solvent-polarity-dependent solution photoluminescence of Au 60 S 6 (SCH 2 Ph) 36 nanoclusters. Not only the maximum emission wavelengths but also the photoluminescence intensities of Au 60 S 6 (SCH 2 Ph) 36 nanoclusters in solution are dependent on the solvent polarity. Note: the excitation wavelength λ ex =514 nm. Full size image In summary, a novel near-infrared-emissive gold nanocluster was synthesized via a thermal-induced ligand exchange process, and its composition was determined to be Au 60 S 6 (SCH 2 Ph) 36 using ESI-MS and SCXC. SCXC also revealed that the nanocluster consists of one fcc-like Au 20 kernel protected by a pair of Au 20 S 3 (SCH 2 Ph) 18 giant staple motifs, which are larger than the existing staple motifs in structurally resolved gold nanoclusters. In particular, three tetrahedral-coordinate μ 4 -S atoms were found enclosed in every giant staple motif, which challenges the conventional opinion that sulfur in the Au–S interface is always three-coordinate μ 2 -S. Most important of all, a 6HLH crystallographic arrangement was found in the crystal of Au 60 S 6 (SCH 2 Ph) 36 nanoclusters, and this finding also represents an advance in crystallographic packing research since the 4H phase finding in 1979. Interestingly, the 6HLH arrangement gives rise to the obvious loss of solid photoluminescence of amorphous Au 60 S 6 (SCH 2 Ph) 36 , indicating the strong interaction among the uniquely arranged nanoclusters. Another interesting finding is the solvent-polarity-dependent solution photoluminescence of Au 60 S 6 (SCH 2 Ph) 36 nanoclusters. Briefly, this work provides new and exciting views to the structure, Au–S bonding and photoluminescence (including solid state and solution) of gold nanoclusters, and our work is expected to stimulate further research on the structure and properties of crystallized materials at the nanoscale. Reagents All chemicals are commercially available and used as received. Tetraoctylammonium bromide (TOAB, 98.0%), 2-Phenylethanethiol (PhC 2 H 4 SH, 99.0%) and phenylmethanethiol (PhCH 2 SH, 99.0%) were purchased from Sigma-Aldrich. Tetrachloroauric(III) acid (HAuCl 4 ·4H 2 O, 99.7%), sodium borohydride (NaBH 4 , 98.0%), acetonitrile (99.0%, AR), dichloromethane (CH 2 Cl 2 , 99.0%, AR), tetrahydrofuran (THF, 99.0%, AR), toluene (99.5%, AR), methanol (CH 3 OH, 99.5%, AR), and petroleum ether (AR) were purchased from Sinopharm Chemical Reagent Co., Ltd. Synthesis of Au 60 S 6 (SCH 2 Ph) 36 nanoclusters All chemicals and reagents were used as received. Ten milligrams of Au 38 (SC 2 H 4 Ph) 24 nanoclusters was dissolved in 1 ml of toluene containing 0.5 ml of PhCH 2 SH. Next, the reaction proceeded overnight at 100 °C under nitrogen atmosphere, and then was terminated by the addition of excess methanol. The crude product was washed with petroleum ether and methanol four times, dissolved in dichloromethane (DCM), and then subjected to separation and purification by PTLC. Single crystals of the purified nanoclusters were grown by the vapour diffusion of acetonitrile into a toluene solution of the purified nanoclusters at 5 °C, and black-coloured crystals formed after one week. Au 38 (SC 2 H 4 Ph) 24 were prepared according to previous reports [44] . Characterization Ultraviolet-visible-near-infrared absorption measurements were performed on a Shimadzu UV-3600 spectrophotometer (DCM as solvent). The single crystal diffraction data of Au 60 S 6 (SCH 2 Ph) 36 was recorded on a Bruker APEXDUO X-ray Diffractometer (Bruker, Germany). ESI-MS was conducted on a Waters Q-TOF mass spectrometer equipped with a Z-spray source, and the source temperature was kept at 70 °C. To prepare the samples for ESI-MS analysis, Au 60 S 6 (SCH 2 Ph) 36 was dissolved in toluene ( ∼ 0.5 mg ml −1 ) and then diluted (1/1, v/v) with an ethanol solution containing 0.5 mM CsOAc. The sample was directly infused into the chamber at 5 μl min −1 . The spray voltage was 2.20 kV, and the cone voltage was kept at 60 V. The solution photoluminescence spectra of Au 60 S 6 (SCH 2 Ph) 36 nanoclusters were recorded on a Fluorolog-3-21, Tempro-01 spectrofluorometer (HORIBA Jobin Yvon), and the excitation wavelength was kept at 514 nm with a slit of 10 nm (OD 514 ∼ 0.047, measured by Ultraviolet-visible-near-infrared spectrophotometer). The solid photoluminescence spectra of Au 60 S 6 (SCH 2 Ph) 36 nanoclusters were recorded on a laser confocal scanning Raman/fluorescence scope (HORIBA Jobin Yvon) and laser (514 nm) power is 0.5 mW. The PTLC plates were eluted with DCM/petroleum ether mixture (1/1, v/v) at room temperature under air atmosphere. Data availability The X-ray crystallographic coordinates for structures reported in this article (see Supplementary Table 1 and Supplementary Data 1 ) have been deposited at the Cambridge Crystallographic Data Centre (CCDC), under deposition number CCDC 1526120. The data can be obtained free of charge from the Cambridge Crystallographic Data Centre via www.ccdc.cam.ac.uk/data_request/cif . All other data are available from the authors on reasonable request. How to cite this article: Gan, Z. et al . The fourth crystallographic closest packing unveiled in the gold nanocluster crystal. Nat. Commun. 8, 14739 doi: 10.1038/ncomms14739 (2017). Publisher’s note : Springer Nature remains neutral with regard to jurisdictional claims in published maps and institutional affiliations.